Self-organization of the vesicular stomatitis virus nucleocapsid into a bullet shape The typical bullet shape of Rhabdoviruses is thought to rely on the matrix protein for stabilizing the nucleocapsid coil. Here we scrutinize the morphology of purified and recombinant nucleocapsids of vesicular stomatitis virus in vitro. We elucidate pH and ionic strength conditions for their folding into conical tips and further growth into whole bullets, and provide cryo-electron microscopy reconstructions of the bullet tip and the helical trunk. We address conformational variability of the reconstituted nucleocapsids and the issue of constraints imposed by the binding of matrix protein. Our findings bridge the gap between the isolated nucleoprotein-RNA string in its form of an undulating ribbon, and the tight bullet-shaped virion skeleton. Vesicular stomatitis virus (VSV), a representative of the Mononegavirales order and the prototype Rhabdovirus, encloses a bullet-shaped skeleton made up of a helical trunk topped by a conical tip. The skeleton contains the negative-strand viral RNA coated with the nucleoprotein N. Upon release of the virus into the infected cell, the nucleocapsid unfolds into an inherently disordered ribbon in which the nucleoprotein is thought to protect and stabilize the RNA. From this point on, two key unresolved questions are the mechanism of the ribbon function as a template for viral replication and transcription, and the mechanism of the ribbon-to-bullet transition during virion assembly. For the first question, progress has been achieved, thanks to the capacity of heterologously expressed rhabdoviral nucleoprotein to nonspecifically encapsidate not only long cellular RNAs but also short RNAs that noncovalently close up into N-RNA rings [1] , [2] . In the case of VSV, almost 80% of the rings contain 10 protomers of N [3] , suggesting that the decamer is their low energy form. The atomic structure of this artificially constrained arrangement was solved by X-ray crystallography [2] and provided insights into the structure of the nucleoprotein subunit, the nature of inter-subunit interactions, the mechanism of genome sequestering and the necessity of conformational rearrangements in the nucleoprotein required for access of the viral polymerase into the RNA-binding cleft [2] , [4] . For the second question, cryo-electron microscopy (cryoEM) analysis of the entire virion recently culminated in a 10 Å resolution three-dimensional (3D) reconstruction of the skeleton trunk, where the viral matrix protein M, which role in the nucleocapsid condensation has been under debate since 30 years [5] , [6] , [7] , [8] , bridges consecutive turns of the N-RNA helix [1] . The bullet shape of the N-RNA was thus proposed to rely on the outer helical scaffold of M fixed in an interleaved position between the adjacent turns of N [3] . Here we analyse the polymorphism of purified viral and recombinant N-RNA ( Fig. 1 ), show that it can fold into bullet-shaped structures in the absence of other viral components and provide cryoEM 3D reconstructions of both the tip ( Fig. 2 ) and the trunk ( Fig. 3 ). 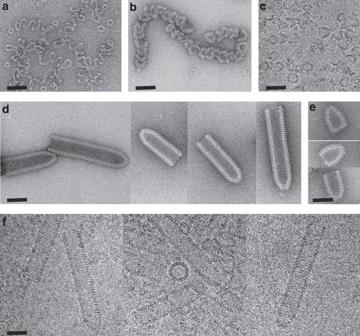Figure 1: VSV N-RNA polymorphism. (a) Loosely coiled N-RNA ribbons (negative stain). (b) Strings of tips (negative stain). (c) Strings of tips (cryoEM). (d) N-RNA bullets (negative stain). (e) N-RNA bullets formed from recombinant VSV N expressed in insect cells and bound to cellular RNA (negative stain). (f) N-RNA bullets (cryoEM). Scale bar, 80 nm ina,b,cand 40 nm ind,e,f. Figure 1: VSV N-RNA polymorphism. ( a ) Loosely coiled N-RNA ribbons (negative stain). ( b ) Strings of tips (negative stain). ( c ) Strings of tips (cryoEM). ( d ) N-RNA bullets (negative stain). ( e ) N-RNA bullets formed from recombinant VSV N expressed in insect cells and bound to cellular RNA (negative stain). ( f ) N-RNA bullets (cryoEM). Scale bar, 80 nm in a , b , c and 40 nm in d , e , f . 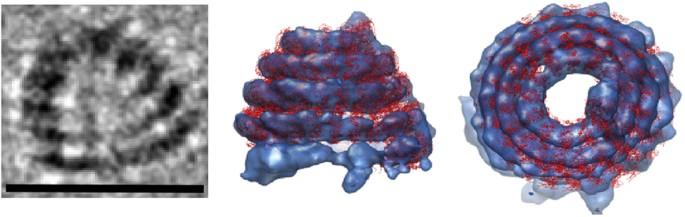Figure 2: CryoEM of N-RNA conical tips. The left panel shows a representative class averages of tips (fromFig. 1c). The middle and the right panels show 3D CryoEM reconstruction of conical tips (blue) with N subunits (red) placed based on the crystal structure of the VSV N-RNA ring deformed to account for the change in tip radius and subunit inclination. Scale bar, 40nm. Full size image Figure 2: CryoEM of N-RNA conical tips. The left panel shows a representative class averages of tips (from Fig. 1c ). The middle and the right panels show 3D CryoEM reconstruction of conical tips (blue) with N subunits (red) placed based on the crystal structure of the VSV N-RNA ring deformed to account for the change in tip radius and subunit inclination. Scale bar, 40nm. 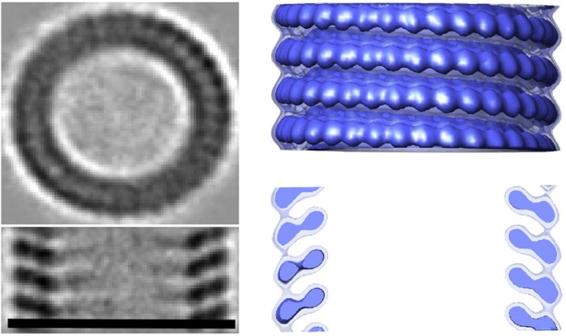Figure 3: CryoEM of the ~33 subunit/turn helical trunk. The left panels show representative class averages of helical trunks (fromFig. 1f, top view of a ~33 subunit/turn bullet and side view). The right panels show the 3D CryoEM reconstruction of the N-RNA bullet trunk and a 20 Å thick central slice through this volume. Scale bar, 40nm. Full size image Figure 3: CryoEM of the ~33 subunit/turn helical trunk. The left panels show representative class averages of helical trunks (from Fig. 1f , top view of a ~33 subunit/turn bullet and side view). The right panels show the 3D CryoEM reconstruction of the N-RNA bullet trunk and a 20 Å thick central slice through this volume. Scale bar, 40nm. Full size image Ribbon-to-tip transition At neutral pH, purified N-RNA forms an undulating ribbon at 150 mM NaCl ( Fig. 1a ) but auto-assembles into a unidirectional necklace of conical tips at low ionic strength ( Fig. 1b ). The tip reconstruction suggests that tip nucleation may start with a 10 subunit-turn compatible with the crystallized recombinant N-RNA decameric rings [2] . The tip features ~5 turns ( Fig. 2 ) with the diameter of the cone’s base reaching ~390 Å. These measures of the in vitro reconstituted N-RNA tips agree with the 450 Å outer diameter of the virion N-RNA trunk proposed to be achieved after ~7 turns [3] . Reconstituted N-RNA bullets Protonation of N at pH 5 and at low ionic strength allows the conical tips to progress into full bullets morphologically similar to the viral skeletons ( Fig. 1d ). The distribution of trunk diameters illustrates their flexibility and ranges from 370 to 415 Å while centred at ~390 Å consistent with the five-turn tips ( Fig. 4 ). Assuming that the dihedral angle between adjacent nucleoprotein subunits in the reconstituted bullets corresponds to the one in the virion, one can then approximate that the in vitro N-RNA bullet trunks contain between ~31 and ~35 subunits per turn as opposed to 37.5 subunits per turn determined for the virion skeleton [3] . An ~25 Å resolution 3D reconstruction of the ~390 Å diameter set contains about 33 N subunits per turn in agreement with estimations based on observed top views ( Fig. 3 ). 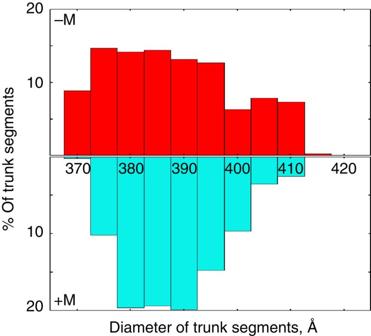Figure 4: Histograms of diameter distribution for the trunk segments. The upper panel shows the diameter distribution of the N-RNA helical trunks in the absence of M (red), the lower in the presence of M (turquoise). Figure 4: Histograms of diameter distribution for the trunk segments. The upper panel shows the diameter distribution of the N-RNA helical trunks in the absence of M (red), the lower in the presence of M (turquoise). Full size image Decoration with the matrix protein M The demonstrated conformational variability and/or flexibility of the reconstituted N-RNA bullets, in particular in terms of their diameter and exact helical symmetry ( Fig. 4 ), indicates that the role of the outer scaffold of M in the VSV skeleton might be to rigidify the nucleocapsid, fixing it precisely at 37.5 subunits per turn as in the cryoEM reconstruction of the virion bullet trunk [3] . Hindered by the previously described self-polymerization of the matrix protein [9] , only partial decoration of the N-RNA bullets by M could be achieved in vitro . At pH 5, addition of M to nucleocapsids ( Supplementary Fig. S1 ) tightens the N-RNA diameter distribution without modifying the global subunit arrangement ( Fig. 4 ; Supplementary Fig. S2 ). The polymorphism of the VSV nucleocapsid, and in particular the ribbon-to-tip and the tip-to-trunk transitions can be considered in the light of the quasi-equivalence concept conceived for capsid proteins of icosahedral viruses [10] and expanded to helical arrangements [11] . Quasi-equivalent subunit assembly is thought to be based on molecular switches that include environment-sensitive elements and are often comprised of disordered segments at subunit interfaces [12] . Here we highlight the role of electrostatic interactions both in the tip nucleation at neutral pH and in the tip-to-trunk transition, probably triggered by neutralization of carboxyl clusters at low pH. We show that bullet formation relies neither on minor viral contaminants nor on the viral RNA but on the nucleoprotein alone, because it takes place no matter if the N-RNA is purified from virus or if the nucleoprotein is expressed in insect cells ( Fig. 1d ) where it binds cellular RNA [12] . The fact that successive nucleoprotein subunits are always tightly arranged along the RNA string, each bound to nine bases of RNA [7] , favours the helical organization of rhabdoviral nucleocapsids by restricting the potentially available conformational space. The proper assembly of icosahedral capsids with large T numbers and of the Mononegavirales nucleocapsids involves auxiliary proteins. The N-RNA of Ebola virus from the filovirus family of Mononegavirales requires the matrix protein for condensation into a flexible helix, further stabilized by additional viral proteins [13] . As for the bullet trunk inside the VSV virion, it is composed of two nested helices: an inner N-RNA helix and an outer M protein helix supposed to confer the bullet shape architecture to the nucleocapsid core [3] , [5] , [6] . Here we show that isolated nucleocapsids can adopt a bullet-shaped structure solely under the effect of pH and ionic strength, and rule out the requirement of other viral components. The outer scaffold of the matrix protein might contribute to rigidification of the bullets restricting them to an exact helical symmetry of 37.5 subunits per turn as observed in the entire virion [3] . The 14-GKKSKK-19 residues of M [14] may have a cementing role at neutral but not at low pH, where the negative charges of N are already neutralized and N-RNA forms bullets on its own. Our study demonstrates that the information necessary for packaging of the VSV genetic material into bullets is contained in the nucleoprotein alone, thus providing a tool for step-by-step analysis of the virion assembly. Biochemical sample preparation N-RNA purification from virus-infected cells . VSV nucleocapsids were isolated from virus-infected cells by CsCl centrifugation as described for rabies virus nucleocapsids [1] . Purified nucleocapsids contained <0.001% of M compared with the M:N ratio in purified virus as determined by western blot analysis. Recombinant N-RNA production in insect cells . cDNA of VSV-N protein of the Indiana laboratory strain (Orsay) originally cloned in a pBluescript II vector [15] , was amplified by PCR and introduced into the pFastBac HTB plasmid, using Rsr II and Xho I restriction sites. The Bac-to-Bac baculovirus (AcMNPV) expression system (Invitrogen) was used to generate recombinant virus. Recombinant nucleocapsids were produced in Spodoptera frugiperda Sf 21 cells and purified by CsCl centrifugation as nucleocapsids isolated from virus. Formation of N-RNA bullets . Immediately before EM analysis, N-RNA samples were extensively dialyzed against MilliQ water at room temperature. The pH of the preparation was then adjusted to 5 or to 7.5 by adding NaAc or Tris-HCl buffer, respectively, up to 5 mM final buffer concentration. Interaction of N-RNA with M and M-N-RNA bullet preparation for EM . VSV M was purified from virus by solubilization with CHAPS as described [9] . Before binding to N-RNA, M protein was subjected to a dialysis against MilliQ water and centrifuged at 80,000 g for 20 min in an Airfuge ultracentrifuge (Beckman Coulter) to remove nucleation sites for self-polymerization. We first tested whether M could bind to N-RNA at both pH 5 and 7 at low salt. For this, N-RNA in 5 mM NaAc pH 5 or 5 mM Tris-HCl pH 7 was incubated with M at 20 °C during 10 min. M was added to N-RNA in a 1:3 M:N-RNA molar ratio. The mixtures (20 μl) were loaded on top of a 15% (v/v) glycerol cushion of 400 μl in the buffer of the binding conditions and centrifuged at 25,000 r.p.m. for 2 h at 20 °C (SW55Ti rotor using Ultra Clear tubes of 0.8 ml). After centrifugation, 20 μl of sample from the top of the glycerol cushion were recovered and the pellet was suspended in 5 μl SDS-PAGE sample buffer. Ten micro litre of each sample was loaded on a 12% SDS-PAGE and proteins were detected by silver staining. Free N-RNA pelleted through the cushion, whereas free M remained at the top. At both pH values M was found in the pellet when mixed with N-RNA ( Supplementary Fig. S1 ). For the EM analysis of the interaction of N-RNA bullets with M, water-dialysed N-RNA and water-dialysed M were mixed at a 1:1 ratio and the pH adjusted to 5 with NaAc buffer (5 mM final buffer concentration). Addition of more M resulted in too much background noise in the EM images. Electron microscopy Negatively stained grids were stained with 2% (w/v) uranyl acetate. For cryoEM, N-RNA was vitrified as described [16] , observed with a Phillips CM200 transmission electron microscope with a LaB 6 filament at 200 kV, and imaged at × 27,500 magnification on Kodak SO-163 films. Negatives were digitized with a Zeiss scanner (Photoscan TD) to a pixel size of 2.55 Å at the specimen level. CryoEM image analysis Image processing was carried out on a Linux cluster. EMAN software [17] was used for particle selection; CTFFIND [18] for contrast transfer function (CTF) determination, BSOFT [19] for the CTF correction; Imagic [20] for multivariate statistical analysis and classification; Spider [21] , [22] for multireference alignment, projection matching (PM) and 3D reconstruction; hsearch and himpose programs from the IHRSR package [23] , [24] for symmetry search and imposition; URO [25] and its graphical version VEDA http://mem.ibs.fr/VEDA , for crystal structure fitting; Pymol [26] and Chimera [27] for visualization. Supplementary Fig. 3 summarizes the flowchart of the image analysis of the helical trunk of the bullet. Two-dimensional image processing Coordinates of the helical trunks’ extremities were recorded with the helix option of the EMAN Boxer tool [17] . Selection of ~1,000 trunks of N-RNA resulted in ~65,000 overlapping 612 × 612 Å segments extracted every 10.2 Å along the trunk axis. The original in-plane angle and filament assignment of the images were recorded for further alignment validation [28] . Individual images were corrected for CTF by phase-flipping, low-pass filtered to 15 Å, normalized (mean=0; sigma=1) and masked by an accordingly rotated smooth-edged rectangular mask of 200 × 560 Å. A vertical version of these images was created for classification. The vertical masked images were iteratively aligned perpendicularly to the helical axis, classified and the eigenvector describing the variability in diameter used for separation of the initial data set into subsets of different diameters of 390±40 Å ( Fig. 4 ). For further analysis, a subset of ~20,000 images was obtained by merging classes with diameters of 390±5 Å. 3D reconstruction First trials of hsearch and himpose did not converge and were very sensitive to parameters of initial symmetry and symmetry search. We therefore started without any symmetry constraints. A smooth and continuous helix of the pitch determined from the class averages was used as a starting model for PM. The first cycle improved the filament boxing in the direction perpendicular to the helical axis by shifting the images by the integer number of pixels closest to the translation value determined by PM. In subsequent PM cycles, this boxing was repeated when translations significantly deviated from zero. The images that could not be unambiguously centred were discarded. This rigorous centring procedure was crucial for minimization of the translational search range during PM, which prevents images from alignment with references requiring too large a translation parallel to helical axis (which in turn can cause clustering of image distribution to certain references thus leading to more and more asymmetric 3D reconstructions). For the same purpose, the same number of images per on-axis view was selected for reconstructions after each PM cycle. Cross-correlation-based selection and other standard single particle-based selection procedures that impose alignment restrains were applied [28] . After ~20 cycles, individual subunits were clearly distinguishable ( Supplementary Fig. S2b ) and the helical symmetry could be visually assessed as ~33 subunits per turn consistent with the rotational symmetry determination of the top view class averages ( Fig. 3 ) and with estimations based on the entire virion nucleocapsid diameter and symmetry. The stacking of the N subunits in subsequent turns appeared quasi vertical. Approximately 12,000 segments of N-RNA were included in the final reconstruction. The PM-reconstruction cycling was then supplemented with a step of refining (hsearch) and imposing (himpose) the symmetry after each iteration. The symmetry parameters converged to 32.8 subunits per turn. The final reconstruction including ~6,000 images of N-RNA was filtered to 22 Å ( Fig. 3 ; Supplementary Fig. S2a ). Analysis of M-N-RNA images and 3D Reconstruction without symmetry application The methodology was the same as for the N-RNA alone. From ~1,000 trunks and ~80,000 initially selected segments of M-N-RNA, ~20,000 segments were included in the final reconstruction obtained without any symmetry constraints, which converged to ~32 subunits per turn for the M-N-RNA complex ( Supplementary Fig. S2c ). Contrary to the N-RNA reconstruction, in the case of M-N-RNA additional stripes of density were noticed all around the map and always at the same distance to the nucleoprotein helix. Comparison with the skeleton in the intact virion [3] indicated that these densities might correspond to the M protein. The relatively low density of M in comparison with the nucleoprotein part can be explained by its non-uniform and non-stoechiometric binding to the nucleoprotein in agreement with the raw images, where the M density was not clearly visible, and with biochemical data on self-polymerization of M [9] . The gap between N and M arises from the Fresnel fringes surrounding the nucleoprotein helix. As the decoration of nucleocapsids by M was clearly substoechiometric, a further symmetry refinement and application seemed inappropriate. Reconstruction of separate bullet tips From negatives binned to 5.1 Å at the specimen level, 6,928 subframes of 128 × 128 pixels containing individual tips were selected, CTF-corrected and low-pass filtered at 15 Å. The data set was translationally but not rotationally aligned relative to the rotationally averaged total sum of the individual images. This translationally centred data set was subjected to multivariate statistical analysis and classification. Representative class averages were examined and circular top views as well as typical side views of the tip containing five prominent striations (as in Fig. 2 ) were identified. Five class averages, which looked most reminiscent of a side view of the tip were each assigned 180 different angles while keeping the views perpendicular to the tube axis. Thus, five crude 3D volumes of the tip were created by back projection and then averaged together to produce a starting model for iterative PM. After ~20 cycles the 3D reconstruction was stable and showed a notable helicity, even if individual N subunits could not be clearly visualized. A total of 4,400 particles were included in the final reconstruction whose resolution was estimated via Fourier shell correlation to be ~40 Å according to the 0.5 criterium. How to cite this article: Ambroise D. et al. Self-organization of the vesicular stomatitis virus nucleocapsid into a bullet shape. Nat. Commun. 4:1429 doi: 10.1038/ncomms2435 (2013).